Large surface relaxation in the organic semiconductor tetracene Organic crystals are likely to have a large degree of structural relaxation near their surfaces because of the weak inter-molecular interactions. The design of organic field-effect transistors requires a detailed knowledge of the surface relaxation as the carriers usually transfer within the first few molecular layers at the semiconductor surfaces, and their transport properties reflect the structural changes through the transfer integral. Here, we report the direct observation of the surface relaxation of an organic semiconductor, a tetracene single crystal, by means of X-ray crystal truncation rod scattering measurements. A significant degree of surface relaxation is observed, taking place only in the first monolayer at the semiconductor surface. First principles calculations show that the resultant transfer integrals are completely different between the bulk and surface of the semiconductor. Crystals have different structures at their surfaces, known as surface relaxation or surface reconstruction. Although they are central issues of surface science, they have less impact on the transport properties of inorganic semiconductors [1] . The surface conductivity originates from the surface-state bands as well as from the bending of the bulk-band, which occurs at the space-charge layer. For surfaces with few adatoms, the former contribution is minor. In the case of organic semiconductors, a significant degree of surface relaxation is likely to occur because of the weak inter-molecular elastic interactions. The resultant self-organized, self-repairing surface layer is expected to have very different electric properties to its bulk counterpart, as the inter-molecular electron transfer is sensitive to the molecular arrangement. If the range of the surface relaxation extends as thick as the space charge layer, the surface transport properties will be completely different from that expected in the bulk. Such surface conductivity is even more important in electronic devices. The application of organic semiconductors in electronic devices has rapidly grown in recent years. Organic electroluminescent displays and organic solar cells are already commercially available. Interfacial charge transfer makes the interface of two insulating organic crystals conductive [2] . In spintronics, organic semiconductors are regarded as attractive materials for use in spin valve devices because of their ability to maintain the spin polarization of the carriers [3] . Most of the functionalities of organic semiconductors are provided by the electron transfer at their interfaces. In fact, the conduction in organic field-effect transistors (OFETs) is confined to the first few molecular layers (~1 nm) at the surfaces [4] when the applied gate electric field is as large as 1 MV cm −1 , which is a normal value for OFETs. Therefore, knowledge of the surface structure of organic semiconductors is essential to understand the microscopic mechanism of the transport properties and to design ideal organic devices with characteristics different from conventional inorganic devices. The attempt to clarify the surface structure is first made in the organic ultra-thin films on SiO 2 substrates [5] , [6] , [7] , which imitate organic thin-film transistors. However, the best performance of organic semiconductors is always found in single crystals. To take advantage of the single crystals, an inkjet printing technique of single-crystal films of organic semiconductors was recently developed [8] . Therefore, the surface of single crystals is of importance. Structural information pertaining to the crystal surface is useful to better understand bulk properties, as the mobility, the standard measure of the performance of an organic semiconductor, is evaluated by fabricating OFETs [9] , [10] , [11] , which is actually the surface mobility [4] . Also, the transport properties in polycrystalline samples are largely affected by scattering at the grain boundaries, which certainly is related to the detail of the interfaces; the knowledge of the surfaces is in fact important as a first step. Recent progress in surface X-ray scattering techniques and analysis methods made it possible to study the details of the surface structure of complicated structured materials. The first observation of the surface structure of organic semiconductor was made on the rubrene single crystal [12] using a combination of X-ray crystal truncation rod (CTR) scattering, which is one of the surface X-ray scattering techniques, and holographic analysis on it [13] . In this study, we perform CTR scattering measurements on tetracene single crystals. The result shows a significant degree of surface relaxation for the first time in the crystalline organic semiconductors, in sharp contrast with rubrene, which hardly shows relaxation. The first principles calculation indeed optimizes such kind of relaxation and shows that the relaxation results in a large modification of the surface band parameters compared with the bulk. The resultant bandwidth and mobility are suppressed in the surface structure. Surface structures of rubrene and tetracene single crystals According to the kinematical theory of X-ray diffraction, the scattering amplitude is given by the Fourier transform of the electron density. The surface is identified as the onset of the zero electron density. Thus, the Fourier transform of the step function is generally observed in scattering from a sample with a flat surface, which is called CTR scattering. The CTR scattering intensity is therefore sensitive to the surface structure and is used to study the structure of the surface. [14] , [15] First, we demonstrate the surface electron density analysis by using rubrene ( Fig. 1f ) single crystal placed on a Si substrate. Figure 2a shows the CTR scattering profile along the (00 L )-line. 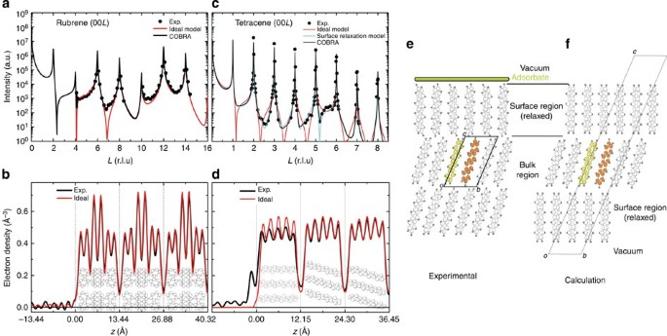Figure 2: Surface structures of the rubrene and tetracene single crystals. (a) The CTR profile of rubrene along the (00L) rod (symbols). The calculated profile for the ideal surface model without relaxation (red curve) is also presented along with the profile for the electron density obtained using COBRA (black curve). (b) The depth dependences of the electron density (ρ(z)) around the nominal surface (z=0). Schematic description of the rubrene molecules with a proper position and size are also shown. The electron density based on the ideal surface model(red line) is shown together. (c,d) Show those for tetracene. The light-blue curve shows the calculated CTR profile for the relaxed surface model after fitting the molecular positions. (e) Schematic of the tetracene surface structure derived from the experimental data. Each unit cell contains two crystallographically inequivalent molecules, indicated in green and orange. (f) An example of the theoretically optimized structure for a free-standing tetracene three-layer. The black circles indicate the experimental results, which all fall on the calculated CTR profile for the ideal surface model. 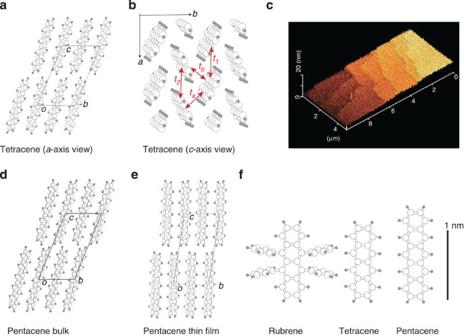Here, the ideal surface model was defined as a surface with no relaxation, reconstruction or roughness. Figure 1: Crystal structures of tetracene and pentacene. The tetracene crystal structure seen from (a) thea-axis and (b) thec-axis. The lattice parameters area=6.075 Å,b=7.93 Å,c=13.46 Å,α=66.6°,β=101°, andγ=94°. The in-plane transfer paths are indicated with arrows. (c) AFM image of a tetracene crystal. (d) the bulk-polymorph structure30(lattice parametersa=6.14 Å,b=7.93 Å,c=16.03 Å,α=67.4°,β=101.9°, andγ=94.2°) and (e) The thin-film-polymorph structure6(lattice parametersa=5.958 Å,b=7.596 Å,c=15.61 Å,α=81.25°,β=86.56°, andγ=89.8°). (f) The molecular structures of rubrene, tetracene and pentacene. Figure 1: Crystal structures of tetracene and pentacene. The tetracene crystal structure seen from ( a ) the a -axis and ( b ) the c -axis. The lattice parameters are a =6.075 Å, b =7.93 Å, c =13.46 Å, α =66.6°, β =101°, and γ =94°. The in-plane transfer paths are indicated with arrows. ( c ) AFM image of a tetracene crystal. ( d ) the bulk-polymorph structure [30] (lattice parameters a =6.14 Å, b =7.93 Å, c =16.03 Å, α =67.4°, β =101.9°, and γ =94.2°) and ( e ) The thin-film-polymorph structure [6] (lattice parameters a =5.958 Å, b =7.596 Å, c =15.61 Å, α =81.25°, β =86.56°, and γ =89.8°). ( f ) The molecular structures of rubrene, tetracene and pentacene. Full size image Figure 2: Surface structures of the rubrene and tetracene single crystals. ( a ) The CTR profile of rubrene along the (00 L ) rod (symbols). The calculated profile for the ideal surface model without relaxation (red curve) is also presented along with the profile for the electron density obtained using COBRA (black curve). ( b ) The depth dependences of the electron density ( ρ ( z )) around the nominal surface ( z =0). Schematic description of the rubrene molecules with a proper position and size are also shown. The electron density based on the ideal surface model(red line) is shown together. ( c , d ) Show those for tetracene. The light-blue curve shows the calculated CTR profile for the relaxed surface model after fitting the molecular positions. ( e ) Schematic of the tetracene surface structure derived from the experimental data. Each unit cell contains two crystallographically inequivalent molecules, indicated in green and orange. ( f ) An example of the theoretically optimized structure for a free-standing tetracene three-layer. Full size image The phase of the scattering amplitude was obtained by a holographic analysis technique called coherent Bragg rod analysis (COBRA) [13] , which we already confirmed to be efficient in the previous study [12] . The CTR amplitude calculated from the ideal surface was used as the reference wave of the hologram to analyse the relaxed surface. Figure 2b shows the electron density profile obtained from the CTR profile in panel (a). The density was averaged over the area of the unit-cell in the c -plane. The observed electron density profile is identical to the profile of the ideal surface model. Therefore, the freshly prepared rubrene crystal exhibits no surface relaxation. The small amount of surface relaxation reported in ref. 12 was caused by degradation of the sample, which occurred during the storage in air. In contrast, we find a large degree of surface relaxation in the tetracene crystals ( Fig. 1a–c ). Figure 2c shows the (00 L )-CTR profile of a tetracene crystal on a Si substrate. The profile was reproduced over three successive measurements, showing that the radiation damage to the sample was negligible. Different pieces of the crystal showed similar intensity profiles, demonstrating that the surface structure of the tetracene crystal in air was stable and reproducible. The same measurements were carried out on a crystal attached to a glass pin, which gave the same CTR profile. This result suggests that the substrate-side of the tetracene surface was either very rough or had the same structure as the air-side of the tetracene surface [16] . The red curve in Fig. 2c shows the profile calculated for an ideal surface, which does not reproduce the experimental results. To develop a surface model that reproduces the experimentally observed CTR profile, a grid search was carried out by translationally shifting the molecules in the first layer, rotating them with respect to the a - and b axes, varying the atomic displacement parameter ( B ) and taking account of the adsorbates. The solid blue curve in Fig. 2c shows the best fit profile. A schematic of the corresponding real space structure is presented in panel (e). Using this structural model as the initial model, electron density analysis was performed using the COBRA method with this CTR profile. Figure 2d shows the electron density profile (the robustness of the resultant profile is examined in the supplementary note 1 and supplementary Fig. 1 ). Here, z =0 was chosen as the nominal surface. The electron density in the z <−3 Å region, which corresponds to outside the sample, is much smaller than that in the crystal. The z > 0 region is divided into molecular layers. From the integrated electron density, each layer at z ≥ 12.15 Å contains 240 electrons per unit cell, the net electron number expected in the bulk crystal. The first molecular layer ranged from 0≤ z ≤12.15 Å and has 237 electrons per unit cell, meaning that there was almost no molecular vacancies in the surface layer. The comparison of the first and the third layers indicates that the surface layer expands by 5.2% along the c -direction. This amount of expansion can be explained by rotating the molecules by 15° about the a -axis. Excess electrons are observed at −3 Å< z < 0 Å, which is attributed to either adsorbates with 18 electrons per unit cell or 37 electrons per nm 2 . Although the present X-ray data do not provide us with the chemical species of the adsorbed matter at the surface, one could anticipate them as being small enough not to deteriorate the basic structure of the surface, and is likely to be water, nitrogen or oxygen molecules. Indeed, the atomic force microscopy measurements in ref. 17 report that the surface of a tetracene crystal has the same in-plane periodicity with the bulk lattice parameters. Our experimental observations pose a question of to what extent the surface relaxation influences the electronic transport properties. Regarding the microscopic charge transport in the accumulation layer in OFETs, the amplitudes of the quantum tunnelling between the highest occupied molecular orbitals (HOMOs), namely the transfer integrals, play a primary role [18] . Therefore, the molecular arrangement is crucial for all of the proposed models ranging from the incoherent hopping to the coherent band-like transport models, which are still under debate. Experimentally, band dispersion measurements by means of photoelectron spectroscopy have been performed on thin films to prevent the charge-up problem [19] , [20] , [21] , and the reports on single-crystal samples are limited [22] , [23] . The theoretical studies on the transport properties reported thus far have been based on bulk single crystals [24] , [25] , [26] , [27] , [28] , [29] . Moreover, none of the studies have taken the surface structure relaxation into account. In our tetracene crystals, the surface relaxation significantly modified the transfer integrals, as demonstrated in the following section. First principles calculations On the basis of the above experimental analysis on tetracene, we performed the first principles electronic structure calculations with the generalized-gradient approximation in the framework of the density functional theory (DFT). The resultant energy bands are shown in Fig. 3 , where a significant difference between the bulk and surface bands can be seen. The transfer integrals along the paths shown in Fig. 1b were calculated using the DFT band structure of the bulk and the surface. The values, together with the effective masses of the holes, are outlined in Table 1 . Although the changes in the effective masses are minor, the transfer integrals t a and t b show large differences. The tight binding energy bands are analytically obtained using the parameters in Table 1 (see Supplementary Note 2 and Supplementary Fig. 2 ). 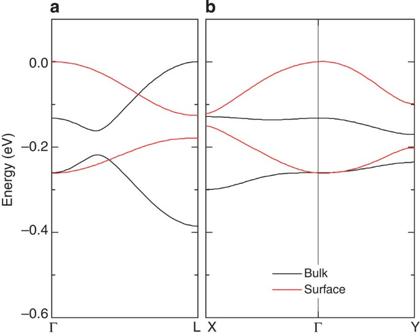Figure 3: In-plane band diagram derived from experimentally obtained bulk and surface structures of tetracene. (a) The band dispersions along the (0,0)-(1/2,1/2) (Γ-L) line. (b) Those along the (1/2,0)-(0,0)-(0,1/2) (X-Γ-Y)line. The origin of the energy is chosen to the valence band maximum. Figure 3: In-plane band diagram derived from experimentally obtained bulk and surface structures of tetracene. ( a ) The band dispersions along the (0,0)-(1/2,1/2) (Γ- L ) line. ( b ) Those along the (1/2,0)-(0,0)-(0,1/2) ( X -Γ- Y )line. The origin of the energy is chosen to the valence band maximum. Full size image Table 1 Transfer integrals of tetracene bulk and surface. Full size table The information on the in-plane structure obtained in the experiments was rather ambiguous compared with that along the direction perpendicular to the surface (see Fig. 2d ). This is because of the experimental difficulty caused by the twinned triclinic crystals having common c *-axis, which hampers the CTR measurements other than (00 L )-line. To compensate for this, we carried out structural optimization of the ‘surface’ layer by putting it on top of a single layer with fixed ‘bulk structure’ obtained in the experiments. We tried several choices of functionals of DFT, finding that, although they showed a large amount of relaxation, the way of relaxing depends quite much on the functionals. The optimized structure of soft organic crystals governed by the van der Waals interactions is often known to deviate quantitatively from the experimental structure. Furthermore, the choice of only a single bulk layer attached to a surface might not be enough to reproduce a real crystal. For these reasons, it is not proper to determine the most suitable relaxed crystal structure solely from the calculations that compare the energies of several candidate structures. Still, we find a reasonable solution that has the similar surface-layer-width with the results of the CTR measurements, which is shown in Fig. 2f . As we see, the angle between the surface and the long molecular axis in the surface molecular layer is closer to 90° than that in the bulk. This situation is similar to the thin film phase pentacene [6] , [30] as presented in Fig. 1d,e . As discussed earlier, the effect of surface relaxation is directly reflected in the large difference of the energy dispersions and in the values of the transfer integrals (see Table 1 ). The HOMO bandwidth of the bulk and the surface are 0.39 and 0.26 eV, respectively, as presented in Fig. 3 . This already indicates that the tetracene surface is less conductive than bulk. To further examine the effect of relaxation on the transport properties, we give a qualitative estimation on the mobility based on these transfer integrals, where we followed the theoretical treatment based on one of the incoherent hopping models [31] . This treatment gives straightforward results, comparable to the experiments and is adopted to the fragment analysis in the DFT-based quantum chemistry calculations. The calculated bulk and the surface mobilities were 1.2 cm 2 V −1 s −1 and 0.3 cm 2 V −1 s −1 at 300 K (see Supplementary Note 3 for details; we used the value of the reorganization energy given in ref. 32 in this calculation). The surface mobility at 300 K was very close to the maximum value of the mobility of tetracene (0.4 cm 2 V −1 s −1 ), which was measured in a high-gate-voltage FET. [11] We should, however, mention that this estimate is at most the semi-quantitative one. There are many other models that are used to determine the mobilities of organic crystals, but discussing the quality of each of the theoretical models is beyond the scope of this study. Still, we would like to argue that the surface relaxation in tetracene makes the surface less conductive by a factor of 1.5 to 3. Now, the two organic semiconductors, rubrene and tetracene, will be compared. The rubrene molecule is obtained by decorating the edges of tetracene molecule with four phenyl substitutions (see Fig. 1f ). The distribution of the HOMOs on these two molecules are almost the same [18] . However, rubrene barely shows a surface relaxation, in sharp contrast to tetracene. This should be because the decorated part of the rubrene molecule works as a structural steric barrier, which does not allow the molecules to tilt freely with respect to the layer. As a result, even though the shapes of HOMOs are the same, the energy band structures and the transport properties represented by the mobility completely differ between the two. This indicates that the choice of the molecular shape should be the key to efficiently controlling the degree of surface relaxation in organic crystals. Finally, a recent report on the photoelectron spectroscopy on rubrene and tetracene single crystals will be discussed [23] . Reference [23] reported a clear band structure of rubrene in agreement with the theoretical prediction [18] , whereas the signal of the HOMO band of the tetracene showed severe broadening, which did not reproduce a reasonable band dispersion. Although they attribute the broadening to the effect of phonon or to the surface disorder, we consider that the latter effect should be small as we find in our X-ray measurement. Our present analysis could instead give another more reasonable scenario; the relaxation taking place only at the single surface layer produces a set of surface energy bands, which significantly differ from the bulk, and the overlap of signals between the surface and the bulk energy bands smears out the details of each of them. This scenario also accounts for the clear dispersion in rubrene, as it has little surface relaxation. In conclusion, CTR scattering measurements are performed on tetracene single crystals and a significant degree of surface relaxation is observed for the first time in organic semiconductors. The details on the molecular structure at the surfaces are clarified by analysing the experimental electron density profile obtained using COBRA, as well as with the first principles calculations. The relaxation is limited to the first molecular layer in the semiconductor, although the relaxed layer is already as thick as the charge accumulation layer in the OFETs, which contributes to the carrier transport. This study clearly demonstrates that the surface relaxation of long-shaped molecules could lead to a qualitative change in its transport properties at the surface. Appropriate design of the molecular structure is the key to controlling the degree of the surface relaxation, which will provide a path to fabricate functional self-organizing surfaces for use in molecular devices. Sample The tetracene crystals were grown by physical vapour transport using a two-zone tube furnace under a continuous stream of Ar gas at a rate of 80 cm 3 min −1 . The diameter of the tube was 20 mm. The upper-stream high-temperature zone was maintained at 220 °C to sublime the tetracene raw materials (sublime grade), purchased from Aldrich Co. The downstream zone was heated to 160 °C to form crystals, typically in 1–2 days. The rubrene crystals were also made in a similar manner. The typical size of the crystals used for the CTR measurements was 2 × 1 mm 2 in area and several micrometres thick. X-ray oscillation photography confirmed that the structures of the tetracene crystals were the same as the one reported in ref. 33 . The lattice parameters used were a =6.075 Å, b =7.93 Å, c =13.46 Å, α =66.6°, β =101° and γ =94°, as shown in Fig. 1a,b . The surface topographies of the crystals were measured with an atomic force microscope (Nanocute, SII nanotechnology) in the dynamic force mode ( Fig. 1c ). Surface X-ray scattering experiments and analyses The CTR scattering experiments were carried out using BL-4C and 3A at the Photon Factory, KEK, Japan. The beamlines are equipped with standard four-circle diffractometers that had a silicon drift detector. X-rays with an energy of 12 keV were used. The spot size was 0.5 × 0.5 mm 2 . All of the experiments were performed in air at room temperature, and the data were collected using transverse scans to subtract the background. Radiation damage to the samples was monitored by repeating the measurements several times. The crystals were placed on Si (001) substrates or attached to glass pins for the CTR measurements. The measurements were performed within a week from the crystal growth. In contrast, in our previous study [12] , the rubrene crystal was kept in air for several months. Coherent Bragg rod analysis was performed using a homemade code with an interpolated experimental data set. As electron density analysis requires a wide q -range of intensity data, the experimental data with calculated intensities below ζ =1.9 and some regions with almost no intensity as well as the regions close to the Bragg reflections were substituted. It was confirmed that the main feature of the electron density was not sensitive to the model used for the substitution, indicating the validity of the analysis method. DFT calculations The ultra-soft pseudopotentials and the plane-wave basis set with cutoff energies of 30 Ry for wavefunctions and 200 Ry for charge densities were used. For the surface band structures, supercell calculations were performed for experimental single-layer structure. The ground state charge densities were computed using 4 × 4 × 2 k -point samplings for the bulk electronic structures, and 4 × 4 × 1 k -points for the surface electronic structures, respectively. To obtain the transfer integrals, we construct a maximally localized Wannier orbital for each tetracene. For the geometry optimization, the system consisting of three molecular layers was considered, with one bulk layer sandwiched between two open surface layers. By assuming the in-plane periodicity of each layer, the structure was optimized with fixing the bulk layer atoms. Such set-up was expected to reproduce the surface relaxation at the two end layers, as the experimental results support that the bulk crystal structure was maintained already at the second layer from the surface. How to cite this article: Morisaki, H. et al. Large surface relaxation in the organic semiconductor tetracene. Nat. Commun. 5:5400 doi: 10.1038/ncomms6400 (2014).